Real-time electrical detection of nitric oxide in biological systems with sub-nanomolar sensitivity Real-time monitoring of nitric oxide concentrations is of central importance for probing the diverse roles of nitric oxide in neurotransmission, cardiovascular systems and immune responses. Here we report a new design of nitric oxide sensors based on hemin-functionalized graphene field-effect transistors. With its single atom thickness and the highest carrier mobility among all materials, graphene holds the promise for unprecedented sensitivity for molecular sensing. The non-covalent functionalization through π–π stacking interaction allows reliable immobilization of hemin molecules on graphene without damaging the graphene lattice to ensure the highly sensitive and specific detection of nitric oxide. Our studies demonstrate that the graphene–hemin sensors can respond rapidly to nitric oxide in physiological environments with a sub-nanomolar sensitivity. Furthermore, in vitro studies show that the graphene–hemin sensors can be used for the detection of nitric oxide released from macrophage cells and endothelial cells, demonstrating their practical functionality in complex biological systems. Nitric oxide (NO) is believed to have diverse and vital roles in neurotransmission, cardiovascular systems and immune responses [1] , [2] . Since NO was first discovered as an elusive endothelial-derived relaxing factor in 1987, extensive research efforts have been devoted to studying the function of NO in physiology and pathology [3] , [4] , [5] . To comprehensively understand the physiological roles of NO and to design new strategies to manipulate NO regulatory pathways for therapeutic purposes, it is desirable to probe the production and diffusion processes of NO in biological systems in real time. To this end, the reliable and specific detection of NO with high spatiotemporal resolution is essential. However, the accurate determination of NO concentration is of significant challenge because of its low concentration (nanomolar scale) and relatively short half-life time (6–50 s) in biological systems [6] , [7] . Indirect detection methods—which rely on sensing secondary species such as nitrite and nitrate—are inherently ineffective for real-time detection. A number of direct detection methods such as electron paramagnetic resonance spectroscopy, chemiluminescence, mass spectrometry and fluorescence [8] , [9] , [10] are being developed for NO detection in biological systems. However, most of these methods either suffer from low sensitivity or require complicated sample preparation or measurement conditions that preclude real-time detection [7] . Electrochemical NO-sensing electrodes allow for real-time detection of NO with high sensitivity and selectivity [11] , [12] , [13] , [14] . However, as the signal amplitude and sensitivity of electrochemical sensors are generally proportional to the electroactive surface area of the electrodes [13] , it is often difficult to simultaneously achieve high sensitivity and high-spatial resolution. Electrochemical NO-sensing electrodes with low nanomolar detection limit usually require an active area of 1,500–30,000 μm 2 (refs 7 , 13 , 14 ), and therefore cannot be used for high-spatial resolution measurements of NO distribution at a single-cell level, which is essential for the understanding of the signal transduction mechanisms of NO in physiology. In addition, electrochemical NO sensors usually operate at a relatively high potential (typically >0.6 V) for the electrochemical oxidation or reduction of NO to occur, which can disturb the intrinsic cellular response or induce significant signal interferences from other electrochemically active molecular species. The application of a coating of NO-selective gas permeable membrane on the electrode can improve the selectivity towards NO. However, greater selectivity usually requires thicker membrane, which not only complicates the fabrication process but also lowers the sensitivity and retards the response speed [7] . With specific molecular functionalization, semiconductor (for example, GaAs)-based field-effect transistors (FETs) can be configured as NO sensors with reduced dimension for real-time detection of NO in physiological solutions [15] . However, the sensitivity of such sensors reported to date is typically limited to the micromolar regime, unsuitable for practical monitoring of biological NO levels that are typically in the nanomolar regime. Nanostructured materials are of increasing interest for the development of highly sensitive chemical and biological sensors [16] , [17] . For example, with the unique single atom thickness and exceptional electrical properties [18] , [19] , [20] , [21] , [22] , [23] , [24] , [25] , graphene has recently received considerable attention for this purpose [26] , [27] , [28] , [29] , [30] , [31] , [32] , [33] , [34] . Here we report the construction of hemin-functionalized graphene FET as a new NO-sensing device for highly sensitive and selective detection of NO in physiological conditions. With the single atom thickness and the highest carrier mobility of all known materials, graphene-based NO sensors hold the promise for exceptional sensitivity that is not possible with other conventional materials for real-time, direct electrical read-out of NO signals. We show that the graphene–hemin sensors can rapidly and selectively respond to NO in physiological solutions with a sub-nanomolar sensitivity, and can be used for real-time monitoring of NO released from macrophage cells and endothelial cells (ECs), demonstrating their practical functionality in complex biological systems. Fabrication and characterization of graphene–hemin sensors Graphene was prepared by mechanical exfoliation onto a silicon substrate with a 300-nm thermal oxide layer. Titanium-gold thin film source, drain and solution gate electrodes were fabricated using e-beam lithography, vacuum metal deposition, followed by a lift-off process. A typical graphene FET device has an active channel area ranging from 0.5 × 0.5 to 0.5 × 2 μm 2 , which is coupled with a polydimethylsiloxane (PDMS) microfluidic channel (with 0.5 mm channel height, 1 mm channel width and 10 mm channel length) for sample delivery ( Fig. 1a ). The graphene FET was non-covalently functionalized with hemin chloride through the π–π stacking interaction to form an NO sensor ( Fig. 1b ) [35] . Hemin is chosen as the functionalization molecule because of its large binding constant and high selectivity towards NO [36] . The non-covalent π–π interaction allows for the functionalization without damaging the graphene lattice or degrading its electronic performance. 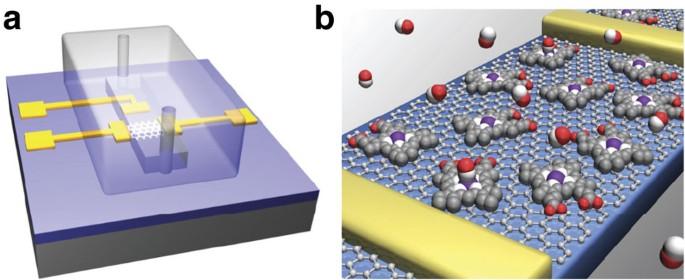Figure 1: Schematic illustration of a graphene–hemin conjugate device. (a) Schematic of a graphene sensor with integrated microfluidic sample delivery system. (b) Schematic illustration of a graphene–hemin FET that can selectively respond to NO. A typical graphene device has an active area of 0.5 × 0.5–0.5 × 2 μm2, sizes of source and drain electrodes are 2 × 5 μm2(excluding the electrical leads) and the size of gate electrode is 50 × 50 μm2. The microfluidic PDMS channel has a width of 1 mm, height of 0.5 mm and length of 1 cm. Figure 1: Schematic illustration of a graphene–hemin conjugate device. ( a ) Schematic of a graphene sensor with integrated microfluidic sample delivery system. ( b ) Schematic illustration of a graphene–hemin FET that can selectively respond to NO. A typical graphene device has an active area of 0.5 × 0.5–0.5 × 2 μm 2 , sizes of source and drain electrodes are 2 × 5 μm 2 (excluding the electrical leads) and the size of gate electrode is 50 × 50 μm 2 . The microfluidic PDMS channel has a width of 1 mm, height of 0.5 mm and length of 1 cm. Full size image Ultraviolet–visible absorption spectroscopy is used to characterize the immobilization of hemin molecules on graphene ( Fig. 2a ). Before hemin functionalization, graphene on quartz only shows expected nearly flat absorption around 2.3% in the visible range (black line in Fig. 2a ). After hemin molecules are conjugated with graphene, a clear absorption peak is observed at 425 nm (red line in Fig. 2a ), close to the Soret band of hemin. The control sample with free hemin in dimethyl sulfoxide (DMSO) solution exhibits an absorption peak at 403 nm (blue line in Fig. 2a ). The red shift of the Soret absorption peak can be attributed to the π–π interaction between graphene and hemin, which rotates the ethylene groups to the coplanar conformation with the porphyrin ring and flattens the hemin molecule to enhance the π conjugation [37] . We have quantified the amount of hemin molecules absorbed on graphene to be 0.94-hemin molecule per square nanometer, nearly a complete monolayer of hemin on graphene (see Supplementary Fig. S1 and Supplementary Note 1 ). 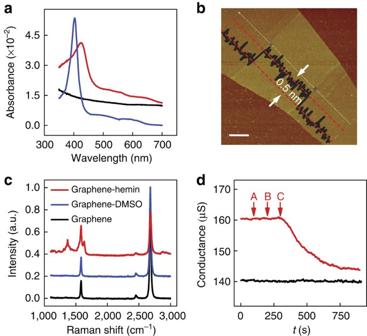Figure 2: Characterization of graphene–hemin conjugate. (a) Ultraviolet–visible spectrum of graphene before and after hemin immobilization. Black: bare graphene; red: graphene after immersed in hemin–DMSO solution, blue: hemin in DMSO solution. (b) AFM image of graphene after hemin immobilization. Scale bar, 1 μm. (c) Raman spectra of graphene before and after hemin functionalization. Black: bare graphene; blue: graphene after immersed in DMSO, with an offset of 0.2; red: graphene–hemin conjugate, with an offset of 0.4. (d) Real-time electrical measurement with NO precursor solution directly added onto a graphene–hemin device inside a PDMS well filled with PBS solution. Graphene–hemin device (red) and bare graphene device (black) were measured in parallel within the same PDMS well. Solution A is 0.01 M NaOH. B is NO precursor in PBS bubbled with N2for 2 h (essentially the same as C but with NO removed). C is NO precursor in NaOH solution (both B and C are 1 μM after diluted in the PDMS well). Figure 2: Characterization of graphene–hemin conjugate. ( a ) Ultraviolet–visible spectrum of graphene before and after hemin immobilization. Black: bare graphene; red: graphene after immersed in hemin–DMSO solution, blue: hemin in DMSO solution. ( b ) AFM image of graphene after hemin immobilization. Scale bar, 1 μm. ( c ) Raman spectra of graphene before and after hemin functionalization. Black: bare graphene; blue: graphene after immersed in DMSO, with an offset of 0.2; red: graphene–hemin conjugate, with an offset of 0.4. ( d ) Real-time electrical measurement with NO precursor solution directly added onto a graphene–hemin device inside a PDMS well filled with PBS solution. Graphene–hemin device (red) and bare graphene device (black) were measured in parallel within the same PDMS well. Solution A is 0.01 M NaOH. B is NO precursor in PBS bubbled with N 2 for 2 h (essentially the same as C but with NO removed). C is NO precursor in NaOH solution (both B and C are 1 μM after diluted in the PDMS well). Full size image Atomic force microscope (AFM) is also used to characterize the hemin-functionalized graphene. To this end, e-beam lithography is used to open up a 3-μm-wide window, where graphene is selectively functionalized with hemin. AFM image of the selectively functionalized graphene shows that the functionalized area exhibits a clear height difference of ~0.5 nm from the unfunctionalized area ( Fig. 2b ), which can be attributed to the formation of a monolayer of hemin molecules on graphene. Raman spectroscopy is used to further characterize the immobilization of hemin molecules on graphene ( Fig. 2c ). The Raman spectrum of bare graphene (black line) shows two main peaks: the G band (1,582 cm −1 ) and the 2D band (2,700 cm −1 ), characteristics of graphene [38] . After hemin functionalization, several new bands are observed at 1,370 cm −1 , 1,631 cm −1 , 1,430 cm −1 and 1,307 cm −1 (red line), which can be assigned for ν 4 , ν 10 , ν 28 and ν 21 vibrational modes of hemin molecules, respectively [39] . A decrease of the 2D band intensity is also observed after hemin immobilization. It was reported that the intensity of the 2D band decreases as a result of the interaction between graphene with either electron-donating or electron-accepting molecules [40] . As a control experiment, a graphene sample is processed in DMSO (the solvent) without hemin through the same procedures of functionalization (blue line). No apparent change is observed in the Raman spectrum compared with the bare graphene before processing, further supporting that the new Raman features (red line) observed in the hemin–graphene conjugate indeed originate from the immobilized hemin on graphene rather than any other processing-induced effects. Hence, these studies clearly demonstrate that hemin molecules are successfully immobilized on graphene. Real-time electrical detection of NO We then tested the electrical responses of graphene devices to NO solutions in real time. All the following real-time electrical measurements were conducted at a constant bias voltage of 10 mV and solution gate of 0 V, unless otherwise stated. The leakage current through the solution gate is typically <3 nA ( Supplementary Fig. S2 ), which is negligible compared with the typical source drain current of the graphene–hemin devices (~1 μA). Two devices on the same substrate were kept in a PDMS well filled with 10 mM phosphate buffered saline (PBS) (pH=7.4), with only one of the devices selectively functionalized with hemin (set-up as in Supplementary Fig. S3 ). Both devices exhibited positive Dirac points with p -type characteristics at 0 V solution gate voltage bias (hole-transport branch). We used diethylamine NONOate sodium as a precursor to release NO in PBS (pH=7.4) [41] , [42] , [43] . At neutral pH, each one of these precursor molecules can hydrolyse to generate two molecules of NO, following a first-order reaction kinetics with a half-life time of ~2 min (ref. 41 ). At basic pH (pH≥12), this hydrolysis reaction proceeds much more slowly and is nearly negligible compared with that at neutral pH. Two devices were tested in parallel. With the introduction of 0.2 μl of a 10 mM NaOH aqueous solution ( Fig. 2d , point A) or 0.2 μl of the precursor/PBS solution, in which NO had been eliminated by 2 h of N 2 bubbling ( Fig. 2d , point B), neither devices showed any obvious conductance change. In contrast, upon the introduction of 0.2 μl of a 100 μM diethylamine NONOate sodium in NaOH solution into the PBS in the PDMS well ( Fig. 2d , point C), the hydrolysis generation of NO is initiated at neutral pH value; the conductance of hemin-functionalized device exhibits a noticeable gradual drop ( Fig. 2d , red line). The time-dependent conductance response curve gives a half-life time of ~135 s, consistent with the hydrolysis kinetics expected for the NO precursor at pH 7.4 (ref. 41 ). On the other hand, the unfunctionalized device does not show any obvious conductance change because there is no active sites for NO binding ( Fig. 2d , black line). This study clearly demonstrates that hemin-functionalized graphene device can indeed respond specifically to NO in PBS solutions. We have further determined the sensitivity of the graphene–hemin NO sensors. To this end, the NO-sensing experiments were performed using a microfluidic system with a PDMS channel integrated on top of the graphene device ( Fig. 1a ), with which the freshly prepared NO solutions of increasing concentrations were introduced into the PDMS channel through a syringe pump. 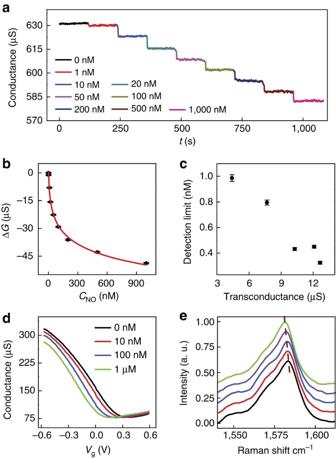Figure 3: Real-time electrical read-out of NO signals. (a) Real-time electrical measurement of different concentrations of NO. (b) Calibration curve: conductance change (ΔG) versus NO concentration (CNO). The red line is the fitted curve in natural logarithmic scale. (c) Relationship of the detection limit versus the transconductance of different sensor devices. (d) Solution gate-dependent measurement at different concentrations of NO.Vg, solution gate voltage. (e) Raman spectra of graphene–hemin in NO solutions at different concentrations. Black: PBS; red: 100 nM NO, with 0.1 offset; blue: 1 μM NO, with 0.2 offset; violet: 10 μM NO, with 0.3 offset; green: 100 μM NO, with 0.4 offset. Figure 3a shows a real-time electrical read-out of different concentrations of NO from 0 to 1,000 nM. The average response time of the steps ( t 90% ) is about 2 s, largely limited by the diffusion at the interface of different concentrations of NO sample solutions (see Supplementary Note 2 ). The inherent response time of the sensor is likely to be much faster. To obtain the calibration curve for NO detection, the amount of the conductance change was plotted against the NO concentration ( Fig. 3b ). The calibration curve in Fig. 3b can be fitted with a logarithmic plot. At low NO background concentration (for example, <10 nM), a lowest absolute detection limit of 0.3 nM can be achieved with a signal-to-noise ratio of 3. With increasing background NO concentration, the absolute sensitivity is reduced. Nonetheless, a relative sensitivity of 3–10% (the percentage of the concentration variation over the background concentration) is maintained consistently even at the highest NO concentration owing to the nature of logarithmic relationship. As the conductance change of the sensor originates from the doping effect, it is expected that the sensor devices with higher transconductance should exhibit higher sensitivity. Indeed, the detection limits of different devices show a consistent trend with a lower detection limit achieved in the device with higher transconductance ( Fig. 3c ). Altogether, these studies clearly demonstrate that the graphene–hemin devices can function as highly sensitive sensors for the detection of NO molecules in PBS. Figure 3: Real-time electrical read-out of NO signals. ( a ) Real-time electrical measurement of different concentrations of NO. ( b ) Calibration curve: conductance change (Δ G ) versus NO concentration ( C NO ). The red line is the fitted curve in natural logarithmic scale. ( c ) Relationship of the detection limit versus the transconductance of different sensor devices. ( d ) Solution gate-dependent measurement at different concentrations of NO. V g , solution gate voltage. ( e ) Raman spectra of graphene–hemin in NO solutions at different concentrations. Black: PBS; red: 100 nM NO, with 0.1 offset; blue: 1 μM NO, with 0.2 offset; violet: 10 μM NO, with 0.3 offset; green: 100 μM NO, with 0.4 offset. Full size image To better understand the effect of NO on the electrical properties of the sensor device, the conductance of the device was plotted against solution gate voltage in PBS with different NO concentrations ( Fig. 3d ). The hemin-immobilized graphene devices show a consistent negative shift of the Dirac point with increasing NO concentration from 0 to 1,000 nM. This negative shift of the Dirac point can be attributed to the doping effect of the hemin complex to the graphene channel upon the binding of NO to the Fe(III) centre. Specifically, with the immobilization of hemin onto graphene, the Fe(III) centre in hemin can interact with graphene in a metal–ligand model, similar to the Fe(III) benzene complexes [44] . In this case, graphene donates π-electrons to the d-orbital of Fe(III) through a cation–π interaction. When NO molecules come to coordinate with and donate electrons to Fe(III) centres, those π-electrons are partially transferred back to the valence band of graphene because of the trans -effect of the ligands [45] . Therefore, the binding of NO to Fe(III) centres is equivalent to partial electron-doping to hemin-functionalized graphene. This electron-doping effect explains the negative shifting of the Dirac point upon the introduction of NO, and is consistent with the reduction of conductance in the hole-transport branch of the graphene devices. Importantly, when monitoring the graphene–hemin device in electron-transport branch, a conductance increase is observed upon the introduction of NO ( Supplementary Fig. S4 ), consistent with the electron-donating nature of the NO-binding events. Raman spectroscopic study was also used to characterize the graphene–hemin device in the PBS solution of NO ( Fig. 3e ). The G band is found to shift to lower frequencies when the NO concentration is increased, consistent with n -type doping to graphene by electron-donating molecules reported in literature [40] . On the other hand, the G band of bare graphene does not exhibit any significant shift of frequency with the increasing NO concentration ( Supplementary Fig. S5 ). It is also important to note that the Raman shift is rather small and only noticeable at relatively high NO concentrations (>100 nM), whereas the electrical signal is detectable at a much lower concentration of NO down to ≤1 nM. Selectivity and functionality in physiological solutions We have further investigated the selectivity and specificity of the graphene–hemin devices as NO sensors. With the introduction of a series of potentially interfering chemicals including oxygen, hydrogen peroxide, sodium nitrate, sodium nitrite, L -citrulline, L -arginine and diethylamine NONOate sodium bubbled with N 2 (which contains only the hydrolysed precursor but not NO), no obvious conductance change is observed ( Fig. 4a ). In contrast, a conductance drop is clearly observed with the addition of 1 nM NO, demonstrating the excellent selectivity of our graphene–hemin NO sensors. We have also tested additional potentially interfering chemicals including L -glutathione, sodium ascorbate, carbon monoxide, hydrogen sulphide, sodium thiocyanate and sodium cyanide with the same devices ( Fig. 4b ). At the same concentration of 100 nM, the device responds to NO with the strongest signal, demonstrating excellent selectivity of our device to NO. 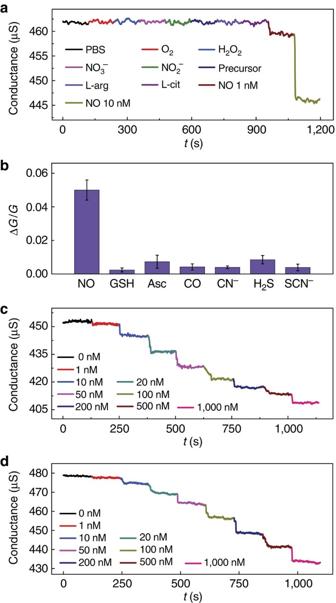Figure 4: Selectivity and practical functionality in physiological solutions. (a) Selectivity measurement with the addition of a series of control solutions (1 μM) followed by NO solutions (1 nM and 10 nM). (b) Selectivity measurement with NO and potentially interfering chemicals (all chemicals have a concentration of 100 nM. GSH,L-glutathione; Asc, sodium ascorbate). Signal is defined by ΔG/G, where ΔGis the conductance change andGis the conductance. The signals are the averages of three devices. (c) Real-time electrical measurement at different concentrations of NO in DMEM. (d) Real-time electrical measurement at different concentrations of NO in fetal bovine serum. Figure 4: Selectivity and practical functionality in physiological solutions. ( a ) Selectivity measurement with the addition of a series of control solutions (1 μM) followed by NO solutions (1 nM and 10 nM). ( b ) Selectivity measurement with NO and potentially interfering chemicals (all chemicals have a concentration of 100 nM. GSH, L -glutathione; Asc, sodium ascorbate). Signal is defined by Δ G / G , where Δ G is the conductance change and G is the conductance. The signals are the averages of three devices. ( c ) Real-time electrical measurement at different concentrations of NO in DMEM. ( d ) Real-time electrical measurement at different concentrations of NO in fetal bovine serum. Full size image To further demonstrate the practical functionality of the sensor in physiological solutions, we have also conducted the NO-sensing measurements in Dulbecco's modified eagle medium (DMEM). The DMEM solution is a typical cell culture medium, containing various kinds of proteins, amino acids, vitamins, inorganic salts and other compounds including glucose. Furthermore, we have also tested the sensor performance in real biological samples such as fetal bovine serum that contains a large variety of potentially interfering species at physiological levels. In both cases, stepwise responses are clearly observed from the NO sensor when different NO concentrations are introduced ( Fig. 4c,d ). Importantly, the detection limits of 0.4 and 1.4 nM were achieved in DMEM solution (see calibration curve shown in Supplementary Fig. S6a ) and fetal bovine serum (see calibration curve shown in Supplementary Fig. S6b ), respectively, demonstrating the proper functionality of our sensors in physiological solutions. We have also evaluated the stability of the graphene–hemin sensors by measuring the sensitivity of the same device after 1 and 3 weeks of storage under ambient conditions ( Supplementary Fig. S7 ). The sensitivity of the sensor is 54 μS per 1,000 nM originally, and became 53 μS per 1,000 nM (98%) after 1 week and 47 μS per 1,000 nM (89%) after 3 weeks, which are comparable to the electrochemical sensors [7] , [12] . This signal drift is probably because of nonspecific surface adsorptions, and the stability of the device may be further improved through storage in a controlled environment. Real-time monitoring of NO released by living cells Going a step further, we have also conducted in vitro studies to test the performance of the graphene–hemin NO sensors for real-time detection of extracellular NO generated from RAW 264.7 macrophage cells. It is well known that macrophage cells can generate NO with expression of inducible NO synthase (iNOS) when stimulated by lipopolysaccharide (LPS) [46] , [47] , [48] , [49] . RAW 264.7 cells were seeded at 5 × 10 5 cells per ml (cell suspension) onto the graphene–hemin device on the SiO 2 substrate (inset, Fig. 5b ) within a PDMS well (set-up as in Supplementary Fig. S3 ). The cells were cultured for 12 h at 37 °C in a 5% CO 2 incubator before NO-sensing measurement. The sensing measurement was carried out at 37 °C. 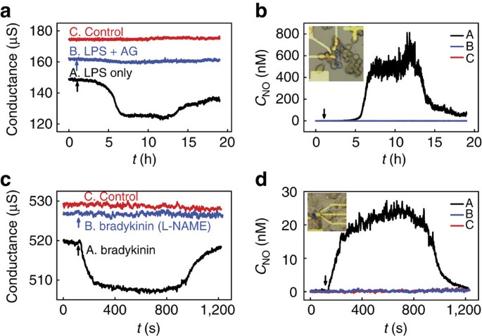Figure 5: Real-time detection of NO released from living cells. (a,b) Real-time monitoring of NO released from Raw 264.7 macrophage cells. (a) Real-time measurement of the conductance of the sensor device for NO detection. (b) Real-time measurement of the NO concentration. Inset: optical microscope image of RAW 264.7 cells seeded on the graphene–hemin device. In both (a,b), (A) 100 ng ml−1LPS, (B) 100 ng ml−1LPS and 100 μM aminoguanidine (AG), (C) without LPS. (c,d) Real-time monitoring of NO released from HUVECs. (c) Real-time measurement of the conductance of the sensor device. (d) Real-time measurement of the NO concentration. Inset: optical microscope image of HUVECs seeded on the graphene–hemin device. In both (c,d), (A) 20 nM bradykinin, (B) 20 nM bradykinin and 1 mML-NG-nitroarginine methyl ester (L-NAME), (C) without bradykinin. Figure 5: Real-time detection of NO released from living cells. ( a , b ) Real-time monitoring of NO released from Raw 264.7 macrophage cells. ( a ) Real-time measurement of the conductance of the sensor device for NO detection. ( b ) Real-time measurement of the NO concentration. Inset: optical microscope image of RAW 264.7 cells seeded on the graphene–hemin device. In both ( a , b ), (A) 100 ng ml −1 LPS, (B) 100 ng ml −1 LPS and 100 μM aminoguanidine (AG), (C) without LPS. ( c , d ) Real-time monitoring of NO released from HUVECs. ( c ) Real-time measurement of the conductance of the sensor device. ( d ) Real-time measurement of the NO concentration. Inset: optical microscope image of HUVECs seeded on the graphene–hemin device. In both ( c , d ), (A) 20 nM bradykinin, (B) 20 nM bradykinin and 1 mM L -NG-nitroarginine methyl ester ( L -NAME), (C) without bradykinin. Full size image As shown in Fig. 5a (A) , after LPS (100 ng ml −1 ) was introduced (at t =1 h), the conductance of graphene–hemin device exhibited a gradual decrease, corresponding to an increase of NO concentration ( Fig. 5b (A) ). The NO concentration reached a maximum around t =6 h and remained stable for the following 5 h, followed by a slow decrease. This time course is consistent with the expected kinetics of NO generation by iNOS in macrophage cells [46] , [47] , [48] . In contrast, when LPS (100 ng ml −1 ) and aminoguanidine (an iNOS inhibitor; 100 μM) were added together, the change of conductance was almost negligible ( Fig. 5a (B) ). The conductance of the control device without LPS stimulation remained as the same value during the measurement ( Fig. 5a (C) ). As shown in Fig. 5b , the conductance of the device was converted to NO concentration by using the calibration curve of the graphene–hemin device ( Supplementary Fig. S8 , red curve). In general, the time response and overall concentration of NO are within the expected ranges for NO generated by macrophage cells. Moreover, the standard Griess test was also used to test NO released by the same batch of RAW 264.7 macrophage cells ( Supplementary Fig. S9 ), which shows a consistent time course with that obtained from the electrical measurements. These results clearly demonstrate that the graphene–hemin sensors are capable of the real-time monitoring of extracellular NO generated from RAW 264.7 macrophage cells over a period of 20 h. Importantly, the calibration curve of the same device after the 20 h of continuous NO measurement shows that the sensitivity of the sensor is largely retained ( Supplementary Fig. S8 ), further demonstrating the excellent long-term stability of the sensor. We have further explored our sensor for the real-time detection of NO released from ECs. The production of NO by vascular ECs has an important role in normal vascular physiology [50] , [51] , [52] . Endothelial-derived NO can account for inhibition of platelet aggregation and adhesion and for the modulation of vascular tone. Direct measurement of NO released from ECs is difficult because NO is generated in small amounts and degrades fast in biological system. Importantly, we show that the graphene–hemin sensor can be readily used to measure NO released by human umbilical vein ECs (HUVECs). The HUVECs were seeded at 5 × 10 5 cells per ml (cell suspension) onto the graphene–hemin device on the SiO 2 substrate (inset, Fig. 5d ) within a PDMS well (set-up as in Supplementary Fig. S3 ). HUVECs were cultured for 12 h at 37 °C in a 5% CO 2 incubator before the NO-sensing measurement. The sensing measurement was carried out at 37 °C. With the introduction of bradykinin (20 nM, an agonist to stimulate the NO generation) at t =120 s, the conductance of graphene–hemin device started to decrease almost instantly ( Fig. ), and reached a plateau after about 150 s. The conductance then kept constant for about 600 s before a gradual increase to almost the original value in about another 200 s. As a control experiment, HUVECs were cultured with culture media with 1 mM L -NG-nitroarginine methyl ester, an endothelial NO synthase inhibitor, for 1 h before the electrical measurement. When bradykinin was added to the control sample, no apparent change of conductance was observed ( Fig. 5c (B) ). The conductance of another control device without bradykinin stimulation kept constant during the measurement ( Fig. 5c (C) ). Using the calibration curve of this graphene–hemin device ( Supplementary Fig. S10 ), the conductance of the device can be converted to NO concentration ( Fig. 5d ). The concentration of NO started to increase after the injection of bradykinin and reached a plateau of ~20 nM in 150 s ( Fig. 5d (A) ). The time course and the concentration of NO are within the expected ranges of NO released by endothelial NO synthase [50] , [51] , [52] . These studies further demonstrate the capability of the graphene–hemin sensors to detect not only large amount of NO over a long period of time but also nanomolar range NO with fast response in complex biological systems. In brief, we have reported a new design of graphene–hemin FET-based NO sensors for direct electrical read-out of NO signals in real time. Unlike electrochemical sensors, the fundamental sensitivities of our graphene NO sensors are not directly dependent on their sizes. It can therefore allow us to scale the sizes of the sensors down to the lithographic limit while retaining high sensitivities. Importantly, our study demonstrates sub-nanomolar detection limit (0.3 nM) can be achieved with submicron graphene–hemin sensors (0.25 μm 2 ), which can only be achieved with electrochemical sensors at least 4–5 orders of magnitude larger (1,500–30,000 μm 2 ). Considering the two-dimensional nature of graphene materials, the miniaturized graphene NO sensor array can be readily integrated over large area for high-spatial resolution detection and imaging of NO signal. In addition, our graphene–hemin NO sensors can operate at a much lower bias voltage (for example, 10 mV) than the working potential of electrochemical NO sensors (for example, >0.6 V), and is therefore less invasive to biological systems. We have shown that the tested NO sensors can exhibit high sensitivity in physiological solutions such as cell culture media or real biological samples such as fetal bovine serum, and can be used for the real-time monitoring of NO released by macrophage cells and ECs. All these samples represent complex real biological conditions with a large number of potentially interfering species at physiological levels. Altogether, these studies clearly demonstrate that our sensors can be used to detect NO in complex biological samples with excellent sensitivity, selectivity, as well as a rapid response speed. Along with their miniaturized sizes, these graphene–hemin NO sensors are promising as a new platform for highly sensitive real-time monitoring of NO signals in biological system with high spatiotemporal resolution. Functionalization of graphene with hemin The graphene devices were immersed in a 1-mg ml −1 hemin chloride/DMSO solution for 2 h to allow the non-covalent functionalization via π–π stacking. The sample was rinsed with DMSO for three times and isopropyl alcohol (IPA) for three times to wash away the unattached hemin molecules. After rinsing with IPA, the sample was blown dry with nitrogen gas. Region selective functionalization The graphene sample was first protected with a layer PMMA and a window was opened using e-beam lithography, and then immersed into hemin/methanol solution for 2 h. The sample was then taken out and rinsed with methanol and IPA. The sample was subsequently immersed in acetone and rinsed with IPA to remove the e-beam resist. Here methanol was used as the solvent to prevent the dissolution of e-beam resist PMMA by DMSO. The sensors functionalized in methanol solution respond to NO the same way as those functionalized in DMSO solution ( Supplementary Fig. S11 ). NO solution preparation NO solution was prepared by dissolving an NO precursor (diethylamine NONOate sodium salt) into 10 mM NaOH solution followed by dilution with 10 mM PBS (pH=7.4), following a protocol developed in previous NO sensor studies [15] . All NaOH and PBS solutions were pre-bubbled with N 2 for 2 h to remove the dissolved oxygen. Diethylamine NONOate sodium salt was added to a 10-mM NaOH solution to make a stock solution of 500 μM. Serial dilution was performed with the stock solution and 10 mM PBS (pH=7.4) to make NO solutions of various concentrations. The NO-containing PBS solutions were allowed to set for at least 15 min before the introduction into the PDMS channel to allow the NO concentrations to saturate. Griess test was used to confirm the concentration of NO generated by diethlyamine NONOate ( Supplementary Fig. S12 ). Device fabrication Graphene was prepared by mechanical exfoliation onto a silicon substrate with a 300-nm thermal oxide layer. Titanium-gold thin film source, drain and solution gate electrodes were formed using e-beam lithography, vacuum metal deposition and a lift-off process. A typical graphene FET device has an active channel area ranging from 0.5 × 0.5 to 0.5 × 2 μm 2 , which is coupled with a PDMS microfluidic channel (with 0.5 mm channel height, 1 mm channel width and 10 mm channel length) for sample delivery. Electrical measurement The electrical transport measurements were conducted with a Lakeshore probe station (Model TTP4) and a computer-controlled analogue-to-digital converter (National Instruments model 6030E). All the sensing measurements were carried out under ambient conditions, with a pre-deposited Ti-Au pad as solution gate electrode. Raw 264.7 cell culture RAW 264.7 cells were obtained from the American Type Culture Collection; ATCC (Manassas, VA, USA) and cultured in DMEM; Carlsbad, CA, USA) containing 10% FCS, 100 U ml −1 penicillin, 100 μg ml −1 streptomycin and 2 mM L -glutamine (complete medium). These cells were maintained in 25 cm 2 cell culture flasks, in which the cells were passaged at 70–80% confluency every 2–4 days. HUVEC culture HUVECs were obtained from the ATCC and cultured in F-12K Medium (ATCC) supplemented with 10% FCS, 0.1 mg ml −1 heparin; 0.05 mg ml −1 EC growth supplement. These cells were maintained in 25 cm 2 cell culture flasks, in which the cells were passaged at 70–80% confluency every 5 days. How to cite this article: Jiang, S. et al . Real-time electrical detection of nitric oxide in biological systems with sub-nanomolar sensitivity. Nat. Commun. 4:2225 doi: 10.1038/ncomms3225 (2013).